The Dishevelled-associating protein Daple controls the non-canonical Wnt/Rac pathway and cell motility Dishevelled is the common mediator of canonical and non-canonical Wnt signalling pathways, which are important for embryonic development, tissue maintenance and cancer progression. In the non-canonical Wnt signalling pathway, the Rho family of small GTPases acting downstream of Dishevelled has essential roles in cell migration. The mechanisms by which the non-canonical Wnt signalling pathway regulates Rac activation remain unknown. Here we show that Daple ( D ishevelled- a ssociating p rotein with a high frequency of leucine residues) regulates Wnt5a-mediated activation of Rac and formation of lamellipodia through interaction with Dishevelled. Daple increases the association of Dishevelled with an isoform of atypical protein kinase C, consequently promoting Rac activation. Accordingly, Daple deficiency impairs migration of fibroblasts and epithelial cells during wound healing in vivo . These findings indicate that Daple interacts with Dishevelled to direct the Dishevelled/protein kinase λ protein complex to activate Rac, which in turn mediates the non-canonical Wnt signalling pathway required for cell migration. Dishevelled (Dvl) is an essential scaffold protein that transduces both the canonical (β-catenin-dependent) and the non-canonical (β-catenin-independent) Wnt signalling pathways [1] , [2] , [3] . In the canonical Wnt signalling pathway, Wnt binding to a receptor complex composed of Frizzled (Fz) and low-density lipoprotein receptor-related protein 5/6 stabilises β-catenin via Dvl, leading to the activation of β-catenin-dependent transcription [4] , [5] , [6] , [7] . It also has been established that Dvl functions in the non-canonical Wnt signalling pathway, which regulates polarised reorganisation of the actin cytoskeleton for cell motility in a β-catenin-independent manner [8] , [9] , [10] . The importance of the non-canonical Wnt signalling pathway has been established in gastrulation movements, dorsoventral patterning, neuronal migration, cochlear hair cell polarity, cardiogenesis and cancer progression [11] , [12] , [13] , [14] , [15] , [16] , [17] , [18] . Previous studies have shown that in the non-canonical Wnt signalling pathway, Dvl activates the Rho family of small GTPases (Rac and Rho), which in turn activates c-jun N-terminal kinase and Rho-associated kinase, respectively [19] , [20] , [21] , [22] . The mechanisms for intracellular signalling in the non-canonical Wnt signalling pathway were revealed, at least partly, by previous studies. Formin-homology protein Daam1 (Dvl-associated activator of morphogenesis-1) interacts with both Dvl and Rho to mediate Wnt-dependent formation of a protein complex of Dvl and Rho, which has pivotal roles in stress fibre formation in HeLa cells and gastrulation movements in Xenopus [8] . In contrast, data are limited regarding the mechanisms by which Wnt induces Rac activation through Dvl, but some clues are available. Studies using Xenopus models and cultured cells suggested that the overexpression of Dvl or Wnt1 stimulation activated Rac through the DEP (Dvl, Egl-10, Pleckstrin) domain of Dvl, which is independent of the Dvl-induced Rho activation mechanisms [8] , [23] . Another study showed that, in cultured hippocampal neurons, the overexpression of Dvl resulted in the activation of Rac, leading to dendritic development [24] . It was also recently shown that Dvl mediates the clathrin-dependent internalisation of the Fz2 receptor in response to Wnt5a, which consequently induces Rac activation [25] . These findings suggest the existence of spatially coordinated regulatory mechanisms of Wnt-dependent Rac activation that are distinct from those of the Rho activation. One candidate protein that links Dvl function to Rac activation is atypical protein kinase C (aPKC; isotypes zeta and lambda/iota), members of the non-classical PKC family [26] . The aPKC is known to be a component of the Par protein complex consisting of three proteins (Par3, Par6 and aPKC), which controls the polarity of epithelial cells and neurons in many organisms [27] , [28] . A previous study showed that Dvl interacts with aPKC to increase the kinase activity of aPKC, which is critical for neuronal polarisation [26] . We previously showed that the Par protein complex mediates Cdc42-induced Rac activation through the recruitment of Rac-specific guanine nucleotide-exchange factors STEF/Tiam1 [29] . Given these findings, it is of interest to ask whether Dvl promotes the activation of Rac through the mobilisation of aPKC and the Par protein complex. A previous yeast two-hybrid analysis identified Daple (Dvl-associating protein with a high frequency of leucine residues) as a novel protein interacting with Dvl [30] . Daple binds to Dvl through its carboxyl terminal (CT) three amino acid residues, which impact the canonical Wnt signalling pathway through the regulation of Tcf transcriptional activity in vitro [30] . Consistent with that observation, Daple negatively regulates the canonical Wnt signalling pathway in Xenopus embryos. The injection of mouse Daple or Xenopus Daple-like protein (termed xDal ) mRNA inhibits Dvl-dependent axis duplication [30] , [31] . The function of Daple is not limited to the regulation of the canonical Wnt signalling pathway. For example, the injection of xDal mRNA in animal pole explants of Xenopus embryos blocked their elongation, which is reminiscent of what is classically observed when the small GTPases Rho or Rac are aberrantly activated in the non-canonical Wnt signalling pathway [31] , [32] . However, it is not understood how Daple regulates the activity of the small GTPases, either in in vitro or in vivo . In this study, we examined the molecular function of Daple using mammalian cells and found that Daple is responsible for the regulation of Dvl-induced activation of Rac, but not other small GTPases in the non-canonical Wnt signalling pathway. Interestingly, Daple induces the formation of the Dvl/PKCλ protein complex to activate Rac, which promotes cell migration. Daple-deficient mice exhibited a defect in skin wound-healing, suggesting a role for Daple in the migration of fibroblasts and epithelial cells in vivo . Thus, Daple/Dvl interaction is important for Rac activation and cell migration, underlining the importance of the Daple/Dvl protein complex in the non-canonical Wnt signalling pathway. Daple enhances the activation of Rac Daple is a large protein with a calculated molecular mass of 226 kDa that possesses a long coiled-coil domain that spans more than two-thirds of the middle of the protein and is flanked on either side by amino terminal (NT) and CT domains ( Fig. 1a,b ). The NT and coiled-coil domains of Daple include the putative oligomerisation domain [30] , [33] . That domain shows close similarities (54%) to that of Girdin, which we recently characterised as an actin-binding protein that promotes cell migration [34] , [35] , [36] , [37] , [38] . Notably, the CT domain of Daple lacks similarities to that of Girdin or any other known functional domain described previously, hinting that the distinctive function of Daple may be located within its CT domain. 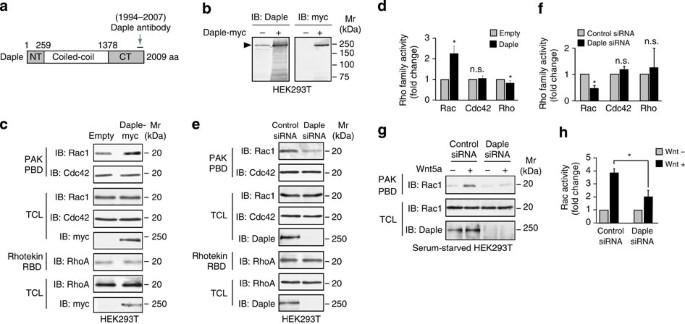Figure 1: Daple regulates the activation of Rac in the non-canonical Wnt signalling pathway. (a) Proposed domain structure of mouse Daple. Daple can be divided into three domains, an N-terminal (NT) domain, a central coiled-coil domain and a CT domain. An arrow indicates the portion of Daple used as an antigen for the production of polyclonal anti-Daple antibody. (b) Endogenous expression of Daple in HEK293T cells shown by western blot analysis (IB) using anti-Daple antibody. The band at 250 kDa detected with anti-Daple antibody corresponded to that detected by anti-myc antibody in myc epitope-tagged Daple (Daple-myc)-transfected cells. (c,d) The activities of Rac, Cdc42 and Rho in HEK293T cell lysates transfected with either control (empty) or Daple-myc were assessed by GST-PAK-PBD or GST-Rhotekin RBD pull-down assays. The precipitates and total cell lysates (TCL) were analysed with the indicated antibodies (c). The intensity of each band for Rac, Cdc42 and Rho was quantified, and the results are presented as fold-induction of the activity of the small GTPases by Daple-myc, compared with the activities in control cells that are expressed as 1.0 (d). (e,f) Activity of Rac, Cdc42 and Rho in HEK293T cell lysates transfected with either control or Daple siRNA. The precipitates and TCL were analysed with the indicated antibodies (e) and quantified (f). (g,h) HEK293T cells transfected with either control or Daple siRNA were stimulated with recombinant Wnt5a (100 ng ml−1) for 1 h. Rac activation was monitored by GST pull-down assays (g). The intensity of each active Rac band was quantified, and the results are presented as the fold-induction of the activity of Rac by Wnt5a, compared with the levels in the absence of Wnt5a that are defined as 1 (h). All bars represent the mean values ±s.d. of three experiments. Significant difference was determined by Student'st-test. *P<0.05, as compared with control cells; n.s., not significant. Figure 1: Daple regulates the activation of Rac in the non-canonical Wnt signalling pathway. (a ) Proposed domain structure of mouse Daple. Daple can be divided into three domains, an N-terminal (NT) domain, a central coiled-coil domain and a CT domain. An arrow indicates the portion of Daple used as an antigen for the production of polyclonal anti-Daple antibody. ( b ) Endogenous expression of Daple in HEK293T cells shown by western blot analysis (IB) using anti-Daple antibody. The band at 250 kDa detected with anti-Daple antibody corresponded to that detected by anti-myc antibody in myc epitope-tagged Daple (Daple-myc)-transfected cells. ( c , d ) The activities of Rac, Cdc42 and Rho in HEK293T cell lysates transfected with either control (empty) or Daple-myc were assessed by GST-PAK-PBD or GST-Rhotekin RBD pull-down assays. The precipitates and total cell lysates (TCL) were analysed with the indicated antibodies ( c ). The intensity of each band for Rac, Cdc42 and Rho was quantified, and the results are presented as fold-induction of the activity of the small GTPases by Daple-myc, compared with the activities in control cells that are expressed as 1.0 ( d ). ( e , f ) Activity of Rac, Cdc42 and Rho in HEK293T cell lysates transfected with either control or Daple siRNA. The precipitates and TCL were analysed with the indicated antibodies ( e ) and quantified ( f ). ( g , h ) HEK293T cells transfected with either control or Daple siRNA were stimulated with recombinant Wnt5a (100 ng ml −1 ) for 1 h. Rac activation was monitored by GST pull-down assays ( g ). The intensity of each active Rac band was quantified, and the results are presented as the fold-induction of the activity of Rac by Wnt5a, compared with the levels in the absence of Wnt5a that are defined as 1 ( h ). All bars represent the mean values ±s.d. of three experiments. Significant difference was determined by Student's t -test. * P <0.05, as compared with control cells; n.s., not significant. Full size image To examine the involvement of Daple in the non-canonical Wnt signalling pathway, we utilised human embryonic kidney HEK293T cells. This line has been used in previous studies to show that exogenous overexpression of the Fz7 receptor and Dvl2 activated both Rac and Rho [8] , [23] . Western blot analyses using anti-Daple antibody showed that Daple was endogenously expressed in HEK293T cells ( Fig. 1b ). Looking at downstream consequences of Daple overexpression in the HEK293T cells, we found that the expression of exogenous myc epitope-tagged Daple more than doubled the active (GTP-binding) form of Rac1, but not those of other small GTPases, RhoA or Cdc42 ( Fig. 1c,d ). In these experiments, it seemed that Rho activity was slightly, but statistically significantly suppressed by the expression of Daple, which may be because of the synergistic inhibitory actions of Rac and Rho [39] . Consistent with this finding, in HEK293T cells that were transfected with Daple-specific small interfering RNA (siRNA) to suppress (knockdown) endogenous Daple, the basal activation level of Rac1 was decreased by about half without significant changes in either RhoA or Cdc42 activation ( Fig. 1e,f ). Specificity of the siRNA for Daple was supported by the observation that two individual siRNA duplexes ( Supplementary Methods ) inhibited Rac activation ( Supplementary Fig. S1a ) and by rescue experiments described later. These data indicate the possibility that Daple specifically regulates the activation of Rac, but not other small GTPases. We next determined whether Daple functions downstream from the non-canonical Wnt signalling pathway. To this end, we utilised Wnt5a, a Wnt ligand protein that is known to signal via the non-canonical Wnt signalling pathway and stimulate the activation of Rac in cultured cells [17] , [25] , [40] . Time-dependent Rac activation induced by Wnt5a was attenuated by the knockdown of Daple ( Fig. 1g,h , Supplementary Fig. S1b ), indicating that Daple functions downstream of Wnt signalling, which is initiated at the cell surface and transmitted to the cytoplasm to control Rac activation. Daple induces Rac activation through its binding with Dvl Next, consistent with the hypothesis that the CT domain of Daple may define its function ( Fig. 1a ), we found that overexpression of the CT domain of Daple (Daple CT; amino acids 1390–2009), but not its NT domain (amino acids 1–259) (data not shown), was sufficient to activate Rac ( Fig. 2a ). Our previous biochemical study mapped the Dvl-interacting region of Daple to the PDZ (PSD-95/Dlg/ZO-1)-binding motif (Gly–Cys–Val) at the end of the CT domain ( Fig. 2b ) [30] . We therefore generated a deletion mutant of Daple CT (Daple CTΔGCV) that lacked the three amino acids that bound Dvl ( Fig. 2b ). Exogenous Daple CTΔGCV, which lost the ability to bind endogenous Dvl2 ( Fig. 2c ), did not induce activation of Rac ( Fig. 2d ). These results suggest that Daple-induced Rac activation was mediated by the binding of Daple to Dvl. Furthermore, we confirmed that the presence of tags on Daple, whether located on the N terminus or C terminus, did not interfere with its interaction with Dvl and Rac activation ( Supplementary Fig. S2a,b ). Those results indicate that the C-terminal region of Daple meets the requirements for binding to the PDZ domain of Dvl, even if it does not contain a free C-terminal end, as observed for other PDZ-binding proteins [41] . 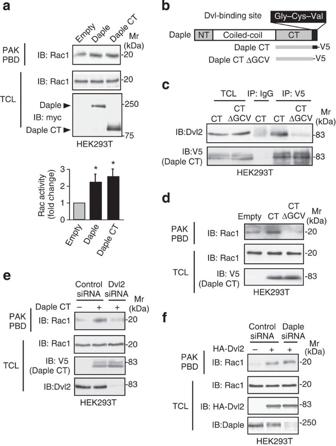Figure 2: Daple induces Rac activation through its binding with Dvl. (a) The activities of Rac in the lysates from HEK293T cells transfected with either control (empty), full-length Daple or CT domain of Daple (Daple CT) were assessed by GST-PAK-PBD pull-down assays. The precipitates and total cell lysates (TCL) were analysed with the indicated antibodies (upper panel) and quantified (lower panel). The results represent the mean values ±s.d. of three experiments. Significant difference was determined by Student'st-test. *P<0.05, as compared with control cells. (b) Schematic illustration of Daple CT tagged with the V5 epitope and its mutant Daple CTΔGCV that lacked the binding site for Dvl. (c) Lysates from HEK293T cells transfected with either Daple CT or Daple CTΔGCV were immunoprecipitated with control IgG or anti-V5 antibody. The precipitates and the TCL were analysed by western blot, using the indicated antibodies. (d) The activities of Rac in lysates from HEK293T cells transfected with either Daple CT or Daple CTΔGCV were assessed by GST-PAK-PBD pull-down assays. (e) The activities of Rac in lysates from HEK293T cells transfected with the indicated combinations of plasmids (control or Daple CT) and siRNAs (control or Dvl2 siRNA) were assessed by GST-PAK-PBD pull-down assays. Daple-CT-induced Rac activation was cancelled by the knockdown of endogenous Dvl2. (f) The activities of Rac in the lysates from HEK293T cells transfected with the indicated combinations of plasmids (control or HA-Dvl2) and siRNAs (control or Daple siRNA) were assessed by GST-PAK-PBD pull-down assays. The precipitates and the TCL were analysed by western blot using the indicated antibodies. Figure 2: Daple induces Rac activation through its binding with Dvl. ( a ) The activities of Rac in the lysates from HEK293T cells transfected with either control (empty), full-length Daple or CT domain of Daple (Daple CT) were assessed by GST-PAK-PBD pull-down assays. The precipitates and total cell lysates (TCL) were analysed with the indicated antibodies (upper panel) and quantified (lower panel). The results represent the mean values ±s.d. of three experiments. Significant difference was determined by Student's t -test. * P <0.05, as compared with control cells. ( b ) Schematic illustration of Daple CT tagged with the V5 epitope and its mutant Daple CTΔGCV that lacked the binding site for Dvl. ( c ) Lysates from HEK293T cells transfected with either Daple CT or Daple CTΔGCV were immunoprecipitated with control IgG or anti-V5 antibody. The precipitates and the TCL were analysed by western blot, using the indicated antibodies. ( d ) The activities of Rac in lysates from HEK293T cells transfected with either Daple CT or Daple CTΔGCV were assessed by GST-PAK-PBD pull-down assays. ( e ) The activities of Rac in lysates from HEK293T cells transfected with the indicated combinations of plasmids (control or Daple CT) and siRNAs (control or Dvl2 siRNA) were assessed by GST-PAK-PBD pull-down assays. Daple-CT-induced Rac activation was cancelled by the knockdown of endogenous Dvl2. ( f ) The activities of Rac in the lysates from HEK293T cells transfected with the indicated combinations of plasmids (control or HA-Dvl2) and siRNAs (control or Daple siRNA) were assessed by GST-PAK-PBD pull-down assays. The precipitates and the TCL were analysed by western blot using the indicated antibodies. Full size image To determine the hierarchy of regulation between Daple and Dvl, siRNAs were used to suppress endogenous Daple and Dvl2, which was reported to potently activate Rac compared with Dvl1 and Dvl3 [23] . Rac activation induced by Daple CT was attenuated by Dvl2 knockdown, whereas the knockdown of Daple did not interfere with exogenously delivered Dvl2-induced Rac activation ( Fig. 2e,f ). These findings indicated the possibility that Daple sits upstream of Dvl in the activation of Rac. Daple facilitates the interaction of Dvl with PKCλ Searching for the mechanism by which Daple activates Rac through its interaction with Dvl, we found that a previously identified interaction between Dvl and aPKC [26] is regulated by Daple ( Fig. 3 ). The overexpression of Daple CT, but not Daple CTΔGCV, augmented the interaction between Dvl and PKCλ, an isoform of aPKC ( Fig. 3a,b ). Consistent with this finding, the knockdown of endogenous Daple attenuated Dvl2/PKCλ interaction ( Fig. 3c ). In those experiments, no interaction between Dvl and PKCζ—a paralogue of PKCλ—was found when a commercially available antibody was used ( Supplementary Fig. S3 ). The results imply a functional difference between the aPKC isoforms, although the experiment does not in itself provide sufficient proof. 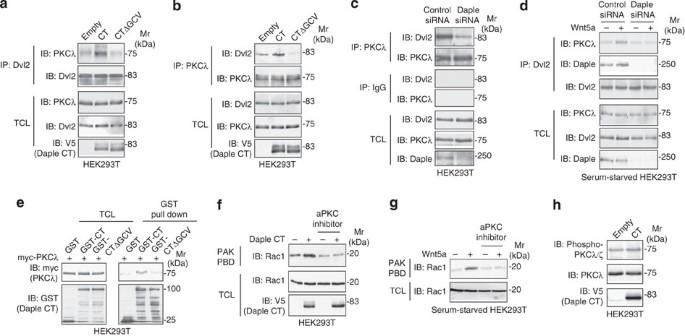Figure 3: Daple regulates the interaction between Dvl and PKCλ in the activation of Rac. (a,b) Lysates from HEK293T cells transfected with control (empty), Daple CT or Daple CTΔGCV were immunoprecipitated with either anti-Dvl2 (a) or anti-PKCλ (b) antibody. The precipitates and the total cell lysates (TCL) were analysed by western blot, using the indicated antibodies. (c) Lysates from HEK293T cells transfected with either control or Daple siRNA were immunoprecipitated with either anti-PKCλ antibody or normal mouse IgG. The precipitates and the TCL were analysed by western blot using the indicated antibodies. (d) Monolayers of confluent HEK293T cells that had been transfected with either control or Daple siRNA were serum-starved for 24 h and stimulated with Wnt5a (100 ng ml−1). The monolayers were wounded and incubated for an additional 30 min. TCL were immunoprecipitated with Dvl2 antibody, followed by western blot analysis using the indicated antibodies. (e) Lysates from HEK293T cells transfected with myc-PKCλ, and either GST, GST-Daple CT, or GST-Daple CTΔGCV were precipitated with glutathione-Sepharose beads. The precipitates and the TCL were analysed by western blot, using the indicated antibodies. (f) HEK293T cells were transfected with either control plasmid or Daple CT, and were incubated in the absence or presence of the aPKC inhibitor, cell-permeable myristoylated aPKC pseudosubstrate, (20 μM) for 1 h. Rac activation was monitored by GST-PAK-PBD pull-down assays. The precipitates and the TCL were analysed by western blot, using the indicated antibodies. (g) HEK293T cells were serum-starved and incubated with Wnt5a either in the absence or presence of the aPKC inhibitor, followed by GST-PAK-PBD pull-down assays to monitor Rac activation. (h) TCL prepared from HEK293T cells transfected with control vector or Daple CT were analysed by western blot, using the indicated antibodies. Figure 3: Daple regulates the interaction between Dvl and PKCλ in the activation of Rac. ( a , b ) Lysates from HEK293T cells transfected with control (empty), Daple CT or Daple CTΔGCV were immunoprecipitated with either anti-Dvl2 ( a ) or anti-PKCλ ( b ) antibody. The precipitates and the total cell lysates (TCL) were analysed by western blot, using the indicated antibodies. ( c ) Lysates from HEK293T cells transfected with either control or Daple siRNA were immunoprecipitated with either anti-PKCλ antibody or normal mouse IgG. The precipitates and the TCL were analysed by western blot using the indicated antibodies. ( d ) Monolayers of confluent HEK293T cells that had been transfected with either control or Daple siRNA were serum-starved for 24 h and stimulated with Wnt5a (100 ng ml −1 ). The monolayers were wounded and incubated for an additional 30 min. TCL were immunoprecipitated with Dvl2 antibody, followed by western blot analysis using the indicated antibodies. ( e ) Lysates from HEK293T cells transfected with myc-PKCλ, and either GST, GST-Daple CT, or GST-Daple CTΔGCV were precipitated with glutathione-Sepharose beads. The precipitates and the TCL were analysed by western blot, using the indicated antibodies. ( f ) HEK293T cells were transfected with either control plasmid or Daple CT, and were incubated in the absence or presence of the aPKC inhibitor, cell-permeable myristoylated aPKC pseudosubstrate, (20 μM) for 1 h. Rac activation was monitored by GST-PAK-PBD pull-down assays. The precipitates and the TCL were analysed by western blot, using the indicated antibodies. ( g ) HEK293T cells were serum-starved and incubated with Wnt5a either in the absence or presence of the aPKC inhibitor, followed by GST-PAK-PBD pull-down assays to monitor Rac activation. ( h ) TCL prepared from HEK293T cells transfected with control vector or Daple CT were analysed by western blot, using the indicated antibodies. Full size image These results were obtained from experiments using HEK293T cells cultured in a nutrient-rich medium containing 10% fetal bovine serum (FBS) lacking the Wnt ligands. However, it is noteworthy that Daple-mediated regulation of Dvl/PKCλ interaction also operated in the non-canonical Wnt signalling pathway. In a confluent monolayer of serum-starved HEK293T cells, Wnt5a stimulation following wounding (to initiate cell migration) promoted Daple/Dvl and Dvl/PKCλ interactions that were effectively suppressed by Daple knockdown ( Fig. 3d ). Formation of the Daple–Dvl–PKCλ tertiary complex was supported by additional GST (glutathione S -transferase) pull-down assays. The results showed that Daple CT, but not the Daple CTΔGCV mutant, interacted with PKCλ ( Fig. 3e ). This was consistent with our previous finding that Daple bound to the PDZ domain, but not other domains of Dvl [30] , suggesting that Daple formed a signalling complex with PKCλ that bound to the DEP domain of Dvl [26] . These data indicated that Daple binding to Dvl is essential for stable formation of the Dvl/PKCλ protein complex to subsequently activate Rac. Importantly, an aPKC-specific inhibitor blocked both Daple CT- and Wnt5a-induced Rac activation ( Fig. 3f,g ). Those data showed that Daple's regulation of Rac activation was dependent on PKCλ kinase activity in the non-canonical Wnt signalling pathway. Further supporting this notion, the expression of Daple CT increased threonine (T) phosphorylation of aPKC in its activation loop (T-403 of PKCλ; T-410 of PKCζ; Fig. 3h ). Daple activates Rac independently of Fz internalisation Given these findings, it was important to understand the mechanism that transmits the signals from the Fz receptor to the Daple/Dvl protein complex in the non-canonical Wnt signalling pathway. Previous studies showed that upon Wnt stimulation, Dvl is recruited to the plasma membrane by the Fz receptor to mediate its clathrin-dependent internalisation [25] . Thus, it seemed possible that Daple acts following the clathrin-dependent internalisation of the Fz receptor. However, neither the overexpression of Fz2 nor Wnt5a stimulation recruited Daple to the plasma membrane ( Supplementary Fig. S4a, b ). These results were consistent with biochemical data that showed that Daple did not coimmunoprecipitate with Fz2 even in the presence of Wnt5a ( Supplementary Fig. S4c ). Also, Daple knockdown did not affect Fz-dependent recruitment of Dvl to the plasma membrane ( Supplementary Fig. S4d ). Taken together, these data suggest that Daple is not involved in the formation of the Fz2/Dvl protein complex at the plasma membrane and its endocytosis. Further supporting this notion, knockdown of the clathrin heavy chain, which effectively suppresses Fz2 internalisation and Wnt5a-induced Rac activation ( Supplementary Fig. S4e ) [26] , failed to suppress Rac activation induced by the overexpression of Daple CT ( Supplementary Fig. S4f ). It is important to note that biochemical fractionation using the lysates prepared from HEK293T cells cultured in the presence or absence of Wnt5a showed that Daple was constitutively present in the membrane fraction ( Supplementary Fig. S4g ). An intriguing but tentative hypothesis is that Daple localises to intracellular membrane-rich organelles such as the endosomes. The precise mode of regulation is unclear at present. However, we speculate that Daple may function to facilitate the formation of the Dvl/PKCλ protein complex on some membrane compartments after, but independently of, the internalisation of the Fz receptor from the plasma membrane. Daple/Dvl interaction regulates the formation of lamellipodia Given that Daple regulates Rac activation and the established role of Rac in reorganisation of polarised actin and the formation of lamellipodia [42] , we examined the effect of Daple overexpression on alterations in cell morphology. In African green monkey kidney (Vero) cells expressing either Daple or Daple CT, but not its mutant Daple CTΔGCV that lacked the ability to activate Rac ( Fig. 2d ), the formation of lamellipodia (which were defined as actin-rich projections greater than 20 μm in width) was more prominent compared with control cells ( Fig. 4a–c ). Conversely, Daple knockdown decreased the basal activation level of Rac and attenuated the formation of lamellipodia in Vero cells ( Fig. 4d–f ). Daple localisation on lamellipodia and the effect of Daple knockdown on cell morphology were also confirmed by staining cells for Cortactin, a lamellipodial marker ( Fig. 4e ). It is of note that the elongation of the cells after Daple knockdown was similar to that observed in human fibroblasts with low Rac activity [43] , further supporting the involvement of Daple in Rac-induced actin reorganisation. We next found that Dvl, whether endogenously or exogenously expressed, colocalised with Daple in the lamellipodia ( Fig. 4g–i , Supplementary Fig. S5 ), indicating that Daple/Dvl interaction is important for the reorganisation of the actin cytoskeleton to form lamellipodia. 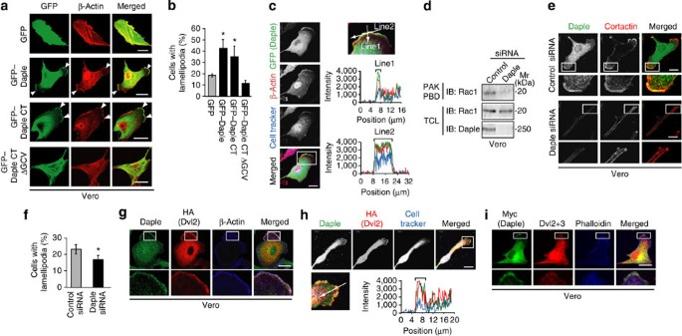Figure 4: Daple/Dvl interaction regulates actin remodelling. (a,b) Expression of Daple and Daple CT, but not Daple CTΔGCV, induced lamellipodia formation in Vero cells cultured in growth medium containing 10% FBS. Arrowheads indicate the lamellipodia (a). The number of cells with lamellipodia was counted in each group and quantified (b). (c) Vero cells transfected with green fluorescent protein (GFP)–Daple were fixed and stained with the indicated antibodies (left panel). The region within the white box is shown at a higher magnification in the right upper panel. Pixel intensities of the green (GFP), red (β-actin) and blue (CMAC) channels were quantified in the sections indicated by Lines 1 and 2 in the right upper panel. The plots indicate pixel intensity (yaxis) over the 15–30 μm sections (xaxis; distance in μm). (d) Vero cells cultured in growth medium containing 10% FBS were transfected with either control or Daple siRNA. The basal activity of Rac was monitored with a GST-PAK-PBD pull-down assay. (e,f) Vero cells transfected with either control or Daple siRNA were fixed and stained with the indicated antibodies. The regions within the white boxes are shown at a higher magnification in adjacent panels. Shown in (f) is the quantification of lamellipodia observed in control and Daple knockdown cells. (g,h) HA-Dvl2-transfected cells were fixed and stained with the indicated antibodies. The regions within the boxes are magnified in the lower panels. Shown in (h) is the quantification of localisation of Daple and Dvl2 at the leading edge. Pixel intensities of the green (Daple), red (Dvl2) and blue (CMAC) channels were quantified in 20-μm sections indicated by an arrow in the left lower panel. (i) Myc-Daple-transfected Vero cells were fixed and stained with the indicated antibodies. For the staining of endogenous Dvls, a cocktail of antibodies containing anti-Dvl2 and anti-Dvl3 was used. The regions within the white boxes are shown at a higher magnification in lower panels. All bars represent the mean values ±s.d. of three experiments. Significant difference was determined by Student'st-test. *P<0.05, as compared with control cells. All scale bars, 20 μm. Figure 4: Daple/Dvl interaction regulates actin remodelling. ( a , b ) Expression of Daple and Daple CT, but not Daple CTΔGCV, induced lamellipodia formation in Vero cells cultured in growth medium containing 10% FBS. Arrowheads indicate the lamellipodia ( a ). The number of cells with lamellipodia was counted in each group and quantified ( b ). ( c ) Vero cells transfected with green fluorescent protein (GFP)–Daple were fixed and stained with the indicated antibodies (left panel). The region within the white box is shown at a higher magnification in the right upper panel. Pixel intensities of the green (GFP), red (β-actin) and blue (CMAC) channels were quantified in the sections indicated by Lines 1 and 2 in the right upper panel. The plots indicate pixel intensity ( y axis) over the 15–30 μm sections ( x axis; distance in μm). ( d ) Vero cells cultured in growth medium containing 10% FBS were transfected with either control or Daple siRNA. The basal activity of Rac was monitored with a GST-PAK-PBD pull-down assay. ( e , f ) Vero cells transfected with either control or Daple siRNA were fixed and stained with the indicated antibodies. The regions within the white boxes are shown at a higher magnification in adjacent panels. Shown in ( f ) is the quantification of lamellipodia observed in control and Daple knockdown cells. ( g , h ) HA-Dvl2-transfected cells were fixed and stained with the indicated antibodies. The regions within the boxes are magnified in the lower panels. Shown in ( h ) is the quantification of localisation of Daple and Dvl2 at the leading edge. Pixel intensities of the green (Daple), red (Dvl2) and blue (CMAC) channels were quantified in 20-μm sections indicated by an arrow in the left lower panel. ( i ) Myc-Daple-transfected Vero cells were fixed and stained with the indicated antibodies. For the staining of endogenous Dvls, a cocktail of antibodies containing anti-Dvl2 and anti-Dvl3 was used. The regions within the white boxes are shown at a higher magnification in lower panels. All bars represent the mean values ±s.d. of three experiments. Significant difference was determined by Student's t -test. * P <0.05, as compared with control cells. All scale bars, 20 μm. Full size image Daple/Dvl interaction regulates cell migration We next ascertained whether the observed localisation of the Daple/Dvl protein complex at the leading edge might be important for cell migration. We found that Daple knockdown cells migrated slower than did control cells in in vitro wound-healing assays ( Fig. 5a,b ). The defect in cell migration in Daple knockdown cells was rescued by the introduction of siRNA-resistant Daple CT, but not its mutant Daple CTΔGCV ( Fig. 5a,b ). In agreement with these results, the decrease in Rac activation in Daple knockdown cells was rescued by siRNA-resistant Daple CT, but not Daple CTΔGCV ( Fig. 5c ). 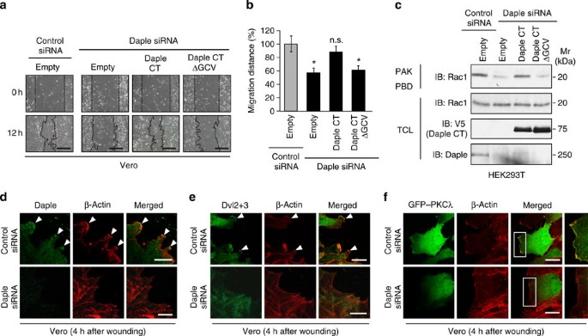Figure 5: Daple/Dvl interaction regulates cell migration. (a,b) Vero cells were transfected with the indicated combination of siRNAs and plasmids, and cultured in growth medium containing 10% FBS. Each monolayer was scratched and incubated for 12 h (a). The wound closure rate was expressed as a ratio of the migration distance in each group divided by the migration distance covered by control cells (b). All bars represent the mean values ±s.d. of three experiments. Significant difference was determined by Student'st-test. *P<0.05 as compared with control (far left bar). Scale bars represent 20 μm. n.s., not significant. (c) HEK293T cells were transfected with the indicated combination of siRNAs and plasmids, followed by GST-PAK-PBD pull-down assays to monitor Rac activation. (d,e) After scratching a monolayer, the cells facing the wound were stained with the indicated antibodies, and images of the leading cells that faced the wound edge were taken by confocal microscopy. Arrowheads indicate the leading edge. Scale bars represent 20 μm. (f) Vero cells were transfected with GFP–PKCλ, and either control or Daple siRNA. After scratching the Vero cell monolayer, cells were fixed and stained with anti-β-actin antibody (red), and images of the leading cells that faced the wound edge were observed. The regions of the leading edge in boxes are magnified in adjacent panels. Scale bars represent 20 μm. Figure 5: Daple/Dvl interaction regulates cell migration. ( a , b ) Vero cells were transfected with the indicated combination of siRNAs and plasmids, and cultured in growth medium containing 10% FBS. Each monolayer was scratched and incubated for 12 h ( a ). The wound closure rate was expressed as a ratio of the migration distance in each group divided by the migration distance covered by control cells ( b ). All bars represent the mean values ±s.d. of three experiments. Significant difference was determined by Student's t -test. * P <0.05 as compared with control (far left bar). Scale bars represent 20 μm. n.s., not significant. ( c ) HEK293T cells were transfected with the indicated combination of siRNAs and plasmids, followed by GST-PAK-PBD pull-down assays to monitor Rac activation. ( d , e ) After scratching a monolayer, the cells facing the wound were stained with the indicated antibodies, and images of the leading cells that faced the wound edge were taken by confocal microscopy. Arrowheads indicate the leading edge. Scale bars represent 20 μm. ( f ) Vero cells were transfected with GFP–PKCλ, and either control or Daple siRNA. After scratching the Vero cell monolayer, cells were fixed and stained with anti-β-actin antibody (red), and images of the leading cells that faced the wound edge were observed. The regions of the leading edge in boxes are magnified in adjacent panels. Scale bars represent 20 μm. Full size image The localisation of Daple, Dvl and PKCλ at the leading edge in migrating cells was abrogated by Daple knockdown, which was accompanied by the loss of prominent lamellipodia ( Fig. 5d–f ). These results indicated that in nutrient-rich medium (containing 10% FBS) without Wnt stimulation, Daple is indeed necessary for spatially controlled localisation of the Dvl/PKCλ protein complex, Rac activation, reorganisation of the actin cytoskeleton and concomitant cell migration. Daple functions in non-canonical Wnt5a-induced cell migration Next, to understand the role of Daple in cell migration mediated by the non-canonical Wnt signalling pathway, we examined the effect of Daple knockdown on Wnt5a-dependent cell migration ( Fig. 6 ). In this experiment, to maximise the effect of Wnt stimulation, we used Vero cells cultured in nutrient-limited medium supplemented with 2% FBS. Consistent with the role of Daple in Wnt5a-induced Rac activation and the formation of the Dvl/PKCλ protein complex ( Figs 1g, h and 3d ), Daple knockdown inhibited cell migration induced by Wnt5a-stimulation ( Fig. 6a, b ). Furthermore, the defect in Wnt5a-dependent cell migration as well as Rac activation in Daple knockdown cells was rescued by the introduction of siRNA-resistant Daple CT, but not its mutant Daple CTΔGCV ( Fig. 6c–e ). These results show the importance of Daple (and its interaction with Dvl) in cell motility that depends on the non-canonical Wnt signalling pathway. It is intriguing (but also a cause for concern) that the data obtained from our haptotaxis migration assays showed that random migration of individual Vero cells was independent of Wnt5a stimulation, regardless of control or Daple knockdown cells ( Supplementary Fig. S6 ). 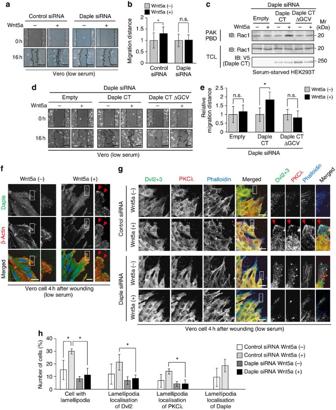Figure 6: Daple regulates Wnt5a-induced lamellipodia formation and cell migration. (a,b) Monolayers of Vero cells transfected with control or Daple siRNA were scratched and incubated in medium supplemented with 2% FBS for 16 h either in the presence (+) or the absence (−) of Wnt5a (a). The wound closure rate was expressed as a ratio of the migration distance in each group divided by that in Wnt5a (−) (b). (c) HEK293T cells transfected with the indicated combination of siRNAs and plasmids were serum-starved for 24 h and stimulated with Wnt5a (100 ng ml−1) for 1 h. Rac activation was monitored by GST pull-down assays. (d,e) Monolayers of Vero cells transfected with the indicated combination of siRNAs and plasmids were scratched and incubated in medium supplemented with 2% FBS in the presence (+) or the absence (−) of Wnt5a for 16 h (d). The wound closure rate was expressed as the ratio of the migration distance (e). (f) Monolayers of Vero cells were scratched, incubated in medium supplemented with 2% FBS in the presence (+) or the absence (−) of Wnt5a for 4 h, and stained with Daple antibody. The leading cells that faced the wound edge are shown. The regions of the leading edge (arrows) in white boxes are magnified in adjacent panels. (g,h) Monolayers of Vero cells transfected with control or Daple siRNA were scratched, incubated in medium supplemented with 2% FBS in the presence (+) or the absence (−) of Wnt5a for 4 h, and stained with the indicated antibodies. The regions of the leading edge (arrows) in white boxes are magnified in adjacent right panels. Shown in (h) are the numbers of cells with lamellipodia and those in which Dvl, PKCλ and Daple are localised at the leading edge in each group. The results are expressed as the percentage of total leading cells. All bars represent the mean values ±s.d. of three experiments. Significant difference was determined by Student'st-test. *P<0.05, between indicated pairs; n.s., not significant. Scale bars represent 300 (a), 100 (d), 20 (f) and 30 μm (g). Figure 6: Daple regulates Wnt5a-induced lamellipodia formation and cell migration. ( a , b ) Monolayers of Vero cells transfected with control or Daple siRNA were scratched and incubated in medium supplemented with 2% FBS for 16 h either in the presence (+) or the absence (−) of Wnt5a ( a ). The wound closure rate was expressed as a ratio of the migration distance in each group divided by that in Wnt5a (−) ( b ). ( c ) HEK293T cells transfected with the indicated combination of siRNAs and plasmids were serum-starved for 24 h and stimulated with Wnt5a (100 ng ml −1 ) for 1 h. Rac activation was monitored by GST pull-down assays. ( d , e ) Monolayers of Vero cells transfected with the indicated combination of siRNAs and plasmids were scratched and incubated in medium supplemented with 2% FBS in the presence (+) or the absence (−) of Wnt5a for 16 h ( d ). The wound closure rate was expressed as the ratio of the migration distance ( e ). ( f ) Monolayers of Vero cells were scratched, incubated in medium supplemented with 2% FBS in the presence (+) or the absence (−) of Wnt5a for 4 h, and stained with Daple antibody. The leading cells that faced the wound edge are shown. The regions of the leading edge (arrows) in white boxes are magnified in adjacent panels. ( g , h ) Monolayers of Vero cells transfected with control or Daple siRNA were scratched, incubated in medium supplemented with 2% FBS in the presence (+) or the absence (−) of Wnt5a for 4 h, and stained with the indicated antibodies. The regions of the leading edge (arrows) in white boxes are magnified in adjacent right panels. Shown in ( h ) are the numbers of cells with lamellipodia and those in which Dvl, PKCλ and Daple are localised at the leading edge in each group. The results are expressed as the percentage of total leading cells. All bars represent the mean values ±s.d. of three experiments. Significant difference was determined by Student's t -test. * P <0.05, between indicated pairs; n.s., not significant. Scale bars represent 300 ( a ), 100 ( d ), 20 ( f ) and 30 μm ( g ). Full size image In wound-healing assays, Wnt5a stimulation promoted the localisation of Daple, Dvl and PKCλ at the leading edge. However, in Daple knockdown cells, the localisation of these proteins at the leading edge was significantly inhibited ( Fig. 6f–h ). Concomitantly, Wnt5a-dependent formation of lamellipodia was significantly inhibited by Daple knockdown. On the basis of these results, we propose a molecular mechanism for Daple-mediated regulation of Rac activation and cell migration in the non-canonical Wnt signalling pathway ( Fig. 7 ). Our findings suggest that Daple facilitates the interaction of Dvl with PKCλ at the leading edge when the cells are stimulated with Wnt5a, thereby promoting Rac activation to regulate actin reorganisation. As indicated above, the involvement of Daple-mediated formation of the Dvl/PKCλ complex in the internalisation of the Fz receptor is unknown at present. 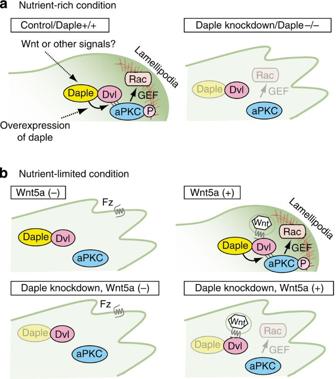Figure 7: A proposed model for Daple-mediated regulation of Rac activation and lamellipodia formation. (a) In cells cultured in nutrient-rich medium (one containing 10% FBS), Daple overexpression facilitates the interaction of Dvl with PKCλ at the leading edge, which results in the activation of Rac and lamellipodia formation. Although speculative at present, it is conceivable that the Dvl/PKCλ protein complex regulates Rac activity through Rac-specific guanine nucleotide-exchange factors (GEFs), such as STEF/Tiam1. It is possible that the serum contains Wnt ligands or alternative external stimuli to promote the function of Daple (left panel). Conversely, Daple depletion attenuates the Dvl/PKCλ complex, leading to the decrease of basal Rac activation (right panel). (b) In cells cultured in nutrient-limited medium or those after serum withdrawal, Wnt5a stimulation induces clathrin-mediated internalisation of the Fz receptor, which signals by recruiting Dvl. Upon Wnt5a stimulation, Daple mediates the formation of the Dvl/PKCλ protein complex, leading to Rac activation and lamellipodia formation (upper panels). Conversely, in Daple-depleted cells, because of the impairment of Dvl/PKCλ interaction, cells fail to activate Rac and form lamellipodia even in the presence of Wnt5a (lower panels). Figure 7: A proposed model for Daple-mediated regulation of Rac activation and lamellipodia formation. ( a ) In cells cultured in nutrient-rich medium (one containing 10% FBS), Daple overexpression facilitates the interaction of Dvl with PKCλ at the leading edge, which results in the activation of Rac and lamellipodia formation. Although speculative at present, it is conceivable that the Dvl/PKCλ protein complex regulates Rac activity through Rac-specific guanine nucleotide-exchange factors (GEFs), such as STEF/Tiam1. It is possible that the serum contains Wnt ligands or alternative external stimuli to promote the function of Daple (left panel). Conversely, Daple depletion attenuates the Dvl/PKCλ complex, leading to the decrease of basal Rac activation (right panel). ( b ) In cells cultured in nutrient-limited medium or those after serum withdrawal, Wnt5a stimulation induces clathrin-mediated internalisation of the Fz receptor, which signals by recruiting Dvl. Upon Wnt5a stimulation, Daple mediates the formation of the Dvl/PKCλ protein complex, leading to Rac activation and lamellipodia formation (upper panels). Conversely, in Daple-depleted cells, because of the impairment of Dvl/PKCλ interaction, cells fail to activate Rac and form lamellipodia even in the presence of Wnt5a (lower panels). Full size image Impaired wound healing in mice with a disrupted Daple gene Finally, to investigate the role of Daple in cell migration in vivo , we generated Daple-deficient mice (Daple −/− ; Supplementary Fig. S7a ). In spite of previous studies showing the effect of Daple manipulation on Xenopus gastrulation [30] , [31] , Daple −/− mice appeared normal upon gross examination of the embryos. Reverse transcription-PCR and western blot analysis showed that Daple expression was increased during embryonic stages and found in nearly all tissues in the early postnatal period ( Supplementary Fig. S7b, c ), indicating compensatory mechanism(s) by other proteins or the possibility that Daple has no obvious role in embryogenesis. However, Daple −/− mice exhibited postnatal weight loss compared with wild-type mice ( Supplementary Fig. S7d ), suggesting the involvement of Daple in the processes that govern cell growth or proliferation, although its precise mechanisms are not known at present. Previous studies showed elevated expression of Wnts in wounded skin and suggested that they contributed to skin wound healing [44] , [45] . Therefore, we evaluated the importance of Daple in cell migration in skin wound-healing assays. Daple −/− mice displayed a significant delay in the closure of excisional wound sites compared with control wild-type mice ( Fig. 8b,c ). Immunohistochemical staining of the skin sections with anti-Daple antibody showed that Daple was highly expressed in wild-type fibroblasts and epithelial cells ( Fig. 8d ). The specificity of the Daple antibody was demonstrated by skin sections prepared from Daple −/− mice ( Fig. 8d ). These findings suggested a role for Daple in the migration of fibroblasts and epithelial cells to promote wound healing. To confirm that the results of the skin wound-healing assay reflected the function of Daple in cell migration, the skin samples of wild-type and Daple −/− mice were separated into fibroblasts and epithelial cells, and the activity of Rac and the migratory response was measured, respectively. As expected, both were attenuated in cells isolated from Daple −/− mice compared with those from wild-type littermates ( Fig. 8e,f ). Consistent with the findings obtained from our experiments using Vero cells ( Fig. 6a,b ), the migration of Daple +/+ fibroblasts cultured in nutrient-limited medium supplemented with 2% FBS was promoted by Wnt5a stimulation. This change was statistically significantly attenuated in Daple −/− fibroblasts ( Fig. 8g,h ). 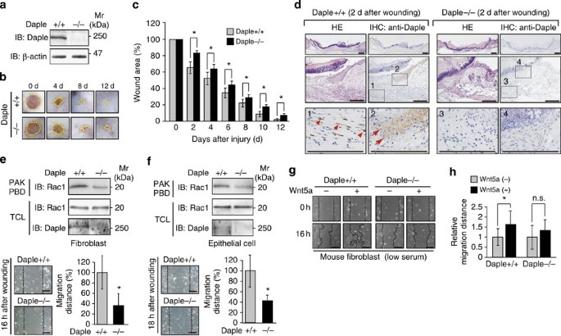Figure 8: Impaired skin wound healing in Daple−/−mice. (a) Western blot analysis of brain lysates from wild-type and Daple−/−P7 mice, using anti-Daple, revealed the absence of Daple in the homozygous mutant mice. (b,c) Wounds were made on the backs of wild-type and Daple−/−P56 mice, and the gross appearance of the wounded areas (dotted lines) was observed for 12 days (b). Wound areas were quantified and expressed as a percentage of the initial wound size (100%) (c). The results represent the mean values±s.e. of six animals. (d) The wound tissue sections prepared from wild-type (left panels) and Daple−/−(right panels) mice 2 days after wounding. The regions in boxes indicate the location of fibroblasts (1, 3) and keratinocytes (2, 4), which are shown at higher magnification in lower panels. Immunostaining with anti-Daple antibody revealed the expression of Daple in fibroblasts (1; arrow heads) and keratinocytes (2; arrows) in the wild-type, but not Daple−/−wound tissues. HE, haematoxylin and eosin; IHC, immunohistochemistry. (e,f) Dermal fibroblasts (e) or epithelial cells (keratinocytes) (f) isolated from skin samples of wild-type and Daple−/−mice were subjected to GST-PAK-PBD pull-down assays (upper panels) and wound-healing assaysin vitro(lower panels). In wound-healing assays, the dotted lines indicate the wound edge at 0 h. The closure rate was expressed as a ratio of the migration distance in each group divided by the migration distance in Daple+/+. Bars represent the mean values ±s.d. of three experiments. (g,h) Fibroblasts harvested from wild-type and Daple−/−mice were incubated in a medium supplemented with 2% FBS. Each monolayer was scratched to induce cell migration in the presence (+) or the absence (−) of Wnt5a, and incubated for 16 h (g). The wound closure rate was expressed as a ratio of the migration distance in each group divided by the migration distance in control (Wnt5a (−)) cells (h). Bars represent the mean values±s.d. of three experiments. Significant difference was determined by Student'st-test. *P<0.05; n.s., not significant. Scale bars represent 200 (d) and 300 μm (e–g). Figure 8: Impaired skin wound healing in Daple −/− mice. ( a ) Western blot analysis of brain lysates from wild-type and Daple −/− P7 mice, using anti-Daple, revealed the absence of Daple in the homozygous mutant mice. ( b , c ) Wounds were made on the backs of wild-type and Daple −/− P56 mice, and the gross appearance of the wounded areas (dotted lines) was observed for 12 days ( b ). Wound areas were quantified and expressed as a percentage of the initial wound size (100%) ( c ). The results represent the mean values±s.e. of six animals. ( d ) The wound tissue sections prepared from wild-type (left panels) and Daple −/− (right panels) mice 2 days after wounding. The regions in boxes indicate the location of fibroblasts (1, 3) and keratinocytes (2, 4), which are shown at higher magnification in lower panels. Immunostaining with anti-Daple antibody revealed the expression of Daple in fibroblasts (1; arrow heads) and keratinocytes (2; arrows) in the wild-type, but not Daple −/− wound tissues. HE, haematoxylin and eosin; IHC, immunohistochemistry. ( e , f ) Dermal fibroblasts ( e ) or epithelial cells (keratinocytes) ( f ) isolated from skin samples of wild-type and Daple −/− mice were subjected to GST-PAK-PBD pull-down assays (upper panels) and wound-healing assays in vitro (lower panels). In wound-healing assays, the dotted lines indicate the wound edge at 0 h. The closure rate was expressed as a ratio of the migration distance in each group divided by the migration distance in Daple +/+ . Bars represent the mean values ±s.d. of three experiments. ( g , h ) Fibroblasts harvested from wild-type and Daple −/− mice were incubated in a medium supplemented with 2% FBS. Each monolayer was scratched to induce cell migration in the presence (+) or the absence (−) of Wnt5a, and incubated for 16 h ( g ). The wound closure rate was expressed as a ratio of the migration distance in each group divided by the migration distance in control (Wnt5a (−)) cells ( h ). Bars represent the mean values±s.d. of three experiments. Significant difference was determined by Student's t -test. * P <0.05; n.s., not significant. Scale bars represent 200 ( d ) and 300 μm ( e – g ). Full size image Despite the identification of many proteins involved in the Wnt signalling pathway, it remains an unsettled and important question how cells regulate Rac activation through Dvl in the non-canonical Wnt signalling pathway [22] , [23] . Here we demonstrated that Daple interacts with Dvl to regulate the formation of Dvl/PKCλ protein complex at the leading edge, leading to Rac activation and cell motility ( Fig. 7 ). We also showed that this signalling cascade is crucial for Wnt5a-induced Rac activation and cell migration ( Fig. 7b ). These findings outline a molecular pathway linking non-canonical Wnt signalling to the activation of Rac in actin remodelling and cell migration. Generally, it has been thought that Dvl proteins serve as a scaffold or hub proteins in the Wnt signalling pathways [1] , [2] , [3] . Daple binds to the PDZ domain, but not the DEP domain of Dvl that interacts with PKCλ and is essential to signal Rac activation. Thus, it is possible that Daple forms a tertiary protein complex with Dvl and PKCλ as ascertained by our biochemical experiments ( Fig. 3a–e ). Given these findings and previous studies that identify many Dvl-interacting proteins, it is plausible to assume that the subcellular localisation and function of Dvl are regulated by its binding proteins such as Daple, which is important to regulate various cellular processes, including cell migration. An important question is how Daple differentially regulates the canonical and non-canonical Wnt signalling pathways. We previously showed that Daple is also involved in the canonical Wnt signalling pathway, where Daple inhibits the accumulation of β-catenin. It appears that this contradicts the stimulatory effect of Daple on the non-canonical Wnt signalling pathway. However, these findings seem to be in accord with previous studies that showed that the non-canonical Wnt signalling pathway antagonises the canonical Wnt signalling pathway [10] , [25] , [46] . A future experimental challenge is to identify cues, which Daple uses in properly controlling its downstream signalling. It was surprising that exogenously added Dvl was able to activate Rac without Daple ( Fig. 2f ), suggesting that Daple sits upstream of Dvl in the non-canonical Wnt signalling pathway. This finding led to the idea that Daple sequesters Dvl at its site of action, thereby stimulating Rac's ability to regulate the reorganisation of the actin cytoskeleton ( Fig. 7 ). This hypothesis was supported by our RNAi experiments that showed that Daple regulates the localisation of Dvl and PKCλ at the leading edge during cell migration ( Figs 4 , 5 and 6 ). Note that experimental conditions are highly relevant in studying how Daple operates in signalling events that take place during cell migration ( Fig. 7a,b ). For example, it is important whether the cells are cultured in a nutrient-rich or -limited (low serum or serum-starved) medium. Our experiments using cells cultured in a low-serum (or serum-deprived) medium clearly demonstrated that Daple and its interaction with Dvl function in Wnt5a-mediated Rac activation and cell migration ( Fig. 7b ). In contrast, but not unexpectedly, Daple regulated Dvl/PKCλ interaction, basal Rac activation and migration in cells cultured with high serum, but in the absence of Wnt ligands ( Fig. 7a ). These results suggest the role of Daple and presumably those of Dvl and aPKC in cell migration that is independent of the non-canonical Wnt signalling pathway ( Fig. 7a ). It remains to be shown which factor(s) other than Wnt5a promotes the formation of the Dvl/PKCλ protein complex through Daple. A related question is how the activity of aPKC, which is required for Daple-mediated Rac activation, is regulated in both nutrient-rich and -limited conditions. At present, it remains unknown how the Dvl/PKCλ protein complex activates Rac downstream of Wnt stimulation. Considering our previous finding that the Par protein complex (that includes aPKC) activates Rac through interaction with Rac-specific guanine nucleotide-exchange factors STEF/Tiam1 [29] , it is possible that the Dvl/PKCλ protein complex uses STEF/Tiam1 to mediate Rac activation. Although our preliminary data suggest a role for Tiam1 in Daple-induced Rac activation (data not shown), further investigation is required to reveal how Daple mobilises Tiam1, and more basically, whether Daple is involved in the Par protein complex. Our study of Daple −/− mice revealed that Daple may participate in cell migration that occurs in postnatal life. Skin wound healing requires the mobilisation and migration of various types of cells to reconfigure normal tissue. This process was attenuated in Daple −/− mice ( Fig. 8 ). However, one concern might be that the effects of Daple deficiency on development are very modest, in comparison with observations obtained from previous studies using Xenopus experimental models [30] , [31] . With regard to this, we should consider compensatory mechanisms in developmental stages. Furthermore, it is of special interest that the function and expression of the non-canonical Wnt proteins are dysregulated in cancer cells [16] , [17] , [18] , and that human Daple/CCDC88C was reported as the prostate cancer risk-associated gene [47] . Therefore, it will be an experimental challenge to investigate the expression and the roles of Daple in the progression of human cancers. Antibodies Rabbit anti-Daple polyclonal antibody was developed against the 14 CT amino acids of Daple (EPGGDPQTVWYEYG) and affinity-purified at a concentration of 2. 2 mg ml −1 as described elsewhere [34] . Anti-phospho-PKCζ/λ, anti-Dvl2 and anti-Dvl3 antibodies were purchased from Cell Signaling Technology (Danvers, MA, USA). Anti-myc and anti-Dvl2 (10B5) antibodies for western blot analysis were purchased from Santa Cruz Biotechnology (Santa Cruz, CA, USA). Other antibodies used in the study include anti-PKCλ antibody (BD Transduction Laboratories, Mississauga, ON, USA), anti-β-actin antibody (Sigma, St Louis, MO, USA), anti-Cortactin antibody (Upstate Biotechnology, Lake Placid, NY, USA), anti-Wnt5a/b (Cell Signaling Technology), anti-clathrin heavy chain and anti-PKCζ antibodies (Santa Cruz), anti-Flag antibody (Sigma), and anti-HA antibody (Roche, Indianapolis, IN, USA). Plasmids A cDNA for mouse Daple that encodes a 2009 amino acid protein was isolated as described previously [30] . The constructs of pcDNA3.1-, pCAG- and pEGFP-Daple fragments, and pEGFP-PKCλ were produced as described elsewhere [34] , [48] . Enhanced green fluorescent protein was fused to the NT, and V5 and myc tags were fused to the CT of the proteins. pCAG-Wnt5a and pCS2-Flag-Fz2 were constructed as described previously [49] . Human Dvl2 cDNA was isolated from HEK293T cells and subcloned into pCGN with an HA tag. The pCAGGS-myc-PKCλ (wild-type and its kinase-dead mutant) plasmids were generously provided by S. Ohno (Yokohama City University, Yokohama, Japan). The target sequences for siRNA-mediated knockdown of Daple was as follow: 5′-TCCAGCTGCGCGTTGTTCAGTGAGG-3′. The knockdown of human Dvl2 expression was done with ON-TARGETplus SMARTpool siRNA (Thermo Scientific, Waltham, MA, USA). Cell lines HEK293T cells and Vero cells were maintained in Dulbecco's modified Eagle's medium supplemented with 10% FBS. HEK293T and Vero cells were transfected with plasmids or siRNA using FuGENE 6 Transfection Reagent (Roche) or Lipofectamine 2000 (Invitrogen). Primary culture of keratinocytes and dermal fibroblasts Full-thickness skin samples from wild-type and Daple −/− P0 mice were incubated in CnT-07 medium (CellnTech, Bern, Switzerland) and 5 mg ml −1 Dispase overnight at 4 °C. The next day, the epidermis and the dermis were separated from the skin sheets and trypsinised to harvest single cells. For Rac activation assays, the keratinocytes were plated on collagen-precoated dishes in serum-free CnT-57 medium at 35 °C. For the wound-healing assay, the monolayers of confluent keratinocytes were scratched in serum-free CnT-02 medium. Dermal fibroblasts were cultured in Dulbecco's modified Eagle's medium supplemented with 15% FBS at 38 °C and used for Rac activation and wound-healing assays. Immunoprecipitation and western blot analysis Cells were lysed in RIPA buffer containing 20 mM Tris-HCl (pH 7.4), 150 mM NaCl, 1 mM EDTA, 1% Triton-X 100, 20 mM β-glycerophosphate and 1 mM p-amidinophenyl methanesulfonyl fluoride hydrochloride supplemented with Complete™ protease inhibitor cocktail (Roche) and PhosSTOP phosphatase inhibitor cocktail (Roche). Lysates were cleared by centrifugation at 12,000× g for 10 min, followed by immunoprecipitation using the indicated antibodies. Samples were separated by SDS-polyacrylamide gel electrophoresis, and proteins were transferred to polyvinylidene difluoride membranes (Millipore, Bedford, MA, USA). Membranes were blocked in 4% milk in PBS containing 0.05% Tween 20, and probed with primary antibodies (1:1000 dilution) and detected by horseradish peroxidase-conjugated secondary antibodies (1:3000 dilution, Dako, Hamburg, Germany). Specific binding was detected with the enhanced chemiluminescence system (Amersham Biosciences, Piscataway, NJ, USA). Rho family small GTPases activation assays Activation of Rac1 and Cdc42 was assayed using a Rac Activation Assay Biochem Kit (Cytoskeleton, Denver, CO, USA). GTP loading of Rac and Cdc42 was determined using Rac/Cdc42 binding domain of Pak1 (p21-activated kinase 1), PAK PBD-GST fusion protein beads according to the manufacturer's protocol. Activation of RhoA was assayed using a Rho Activation Assay Biochem Kit (Cytoskeleton). The amount of PAK PBD/GTP-Rac (or GTP-Cdc42) or Rhotekin RBD/GTP-Rho, which was pulled down was determined by western blot analysis using Rac1-, Cdc42- or RhoA-specific antibodies. Where appropriate, the cells were starved for 16 h, and treated with 100 ng ml −1 recombinant mouse Wnt5a (StemRD, Burlingame, CA, USA) or 20 μM aPKC inhibitor, myristoylated PKCζ pseudosubstrate (Calbiochem, San Diego, CA, USA) for 1 h. GST pull-down assays Daple CT fragments were inserted into the pEF-BOS-GST vector to generate fusion proteins with GST at the NT. HEK293T cells were transfected with GST-Daple CT expression vectors and cultured for 24 h. Cells were then lysed with RIPA buffer and clarified by centrifugation at 12,000× g for 10 min at 4 °C. The soluble supernatant was incubated with glutathione-Sepharose 4B beads (GE Healthcare) for 1 h at 4 °C. The beads were washed with lysis buffer, and their binding proteins were eluted by SDS sample dilution buffer. Aliquots of the eluates were subjected to SDS-polyacrylamide gel electrophoresis, followed by western blot analysis using the indicated antibodies. Immunocytochemistry Cells grown in glass dishes were fixed in 4% (w/v) paraformaldehyde, permeabilised with PBS containing 0.1% (v/v) TritonX-100 and 2% BSA. The cells were incubated with antibodies against Daple, β-actin, Dvl2, Dvl3, HA, myc and PKCλ (1:300 dilution), followed by staining with Alexa 488/594-conjugated goat anti-mouse/rabbit IgG (1:1000 dilution) and Alexa 350-conjugated Phalloidin (1:1000 dilution, Invitrogen). After washing in PBS, fluorescence was visualised by a confocal laser-scanning microscope FLUOVIEW FV500 (Olympus, Tokyo, Japan), followed by quantification of fluorescence in digital images. In the evaluation of localisation of Daple and Dvl at the leading edge, normalised immunofluorescence intensity was evaluated as the ratio of Daple or Dvl fluorescence intensity to cell volume, as measured by the fluorescent signal from Cell Tracker Blue CMAC (chloromethyl derivative of aminocoumarin) (Molecular Probes, Eugene, OR, USA). In the analyses of cell morphology and protein localisation, cells bearing lamellipodia with a width greater than 20 μm were counted as 'cells with lamellipodia'. At least 50 cells were counted per experiment, and the data are presented as the mean values ±s.d. obtained from three independent experiments. Significant difference between Daple and control was determined by Student's t -test. In vitro wound-healing assay Directional cell migration of Vero cells was stimulated in a monolayer by using an in vitro scratch wound assay [50] . Vero cells were transfected with the indicated siRNAs, and seeded on collagen or poly-D-lysine-precoated 35-mm glass dishes after 24 h of transfection. A total of 48 h after the transfection, the confluent Vero cells were scratched with a 200 μl disposable plastic pipette tip and were allowed to migrate towards the wound. To examine Wnt5a-dependent migration in Vero cells, the medium was replaced with that supplemented with 2% FBS either in the presence or absence of Wnt5a, followed by scratching. The cells were fixed at the indicated times for immunofluorescent staining. Wound closure rates were expressed as a percentage of the migratory distance in control cells (100%). In vivo wound-healing assay in Daple knock-out mice Daple knock-out mice were purchased from TransGenic (Kumamoto, Japan). All animal studies were approved by the Animal Care and Use Committee of Nagoya University Graduate School of Medicine. All animal experiments were performed in accordance with the institutional guidelines and regulations. In in vivo wound-healing assays, the backs of mice were shaved and four full-thickness wounds were created on each animal using 4-mm biopsy punches (Kai Industries, Gifu, Japan). Wound sites were digitally photographed at the indicated time intervals, and each wound area was quantified with WinRoof software (Mitani, Fukui, Japan). Wound areas were expressed as a percentage of the initial wound size (100%). Data are presented as means±s.d. Statistical significance was evaluated with Student's t test. Two days after wounding, mice were killed, and rectangular samples of skin containing complete wounds were harvested for histological studies. Histological and immunohistochemical analyses Skin samples were fixed in 10% paraformaldehyde, paraffin-embedded and sectioned at 4 μm for light microscopic analysis. Haematoxylin and eosin staining was performed by conventional methods. The sections were stained with Daple antibody (1:10,000 dilution) using a CSA kit (Dako) according to the manufacturer's recommendations. The specificity of the Daple antibody was determined in an absorption test using an excess amount of the peptide for immunisation. Sections were pretreated by microwaving in citrate buffer for 10 min to retrieve antigenicity. Haematoxylin was used for the counterstaining. Images were taken with an Olympus BX50 microscope (Olympus). Statistical analyses In Rho family small GTPases activation assays, the band intensity of each pull-down sample was normalised to the band of total cell lysate on the same sample, and the ratio for the control sample (empty vector or control siRNA) was arbitrarily set as 'one'. All data are presented as mean values±s.d. from three independent experiments ( n =3). Significant difference was determined by Student's t -test, and P -values less than 0.05 were considered statistically significant. In wound-healing assays, the wound width was measured at five points in each sample, followed by the calculation of migration distance. Data are presented as the ratio of migration distance of each sample to that of control sample (control siRNA or Wnt5a stimulation (−)). All data are presented as mean values±s.d. from three independent experiments. Significant difference was determined by Student's t -test, and P -values less than 0.05 were considered statistically significant. How to cite this article: Ishida-Takagishi, M. et al . The Dishevelled-associating protein Daple controls the non-canonical Wnt/Rac pathway and cell motility. Nat. Commun. 3:859 doi: 10.1038/ncomms1861 (2011).